Diminished hERG K+channel activity facilitates strong human labour contractions but is dysregulated in obese women Human ether-a-go-go-related gene (hERG) potassium channels determine cardiac action potential and contraction duration. Human uterine contractions are underpinned by an action potential that also possesses an initial spike followed by prolonged depolarization. Here we show that hERG channel proteins (α-conducting and β-inhibitory subunits) and hERG currents exist in isolated patch-clamped human myometrial cells. We show that hERG channel activity suppresses contraction amplitude and duration before labour, thereby facilitating quiescence. During established labour, expression of β-inhibitory protein is markedly enhanced, resulting in reduced hERG activity that is associated with an increased duration of uterine action potentials and contractions. Thus, changes in hERG channel activity contribute to electrophysiological mechanisms that produce contractions during labour. We also demonstrate that this system fails in women with elevated BMI, who have enhanced hERG activity as a result of low β-inhibitory protein expression, which likely contributes to the weak contractions and poor labour outcomes observed in many obese women necessitating caesarean delivery. Our poor understanding of the mechanisms regulating the onset and progress of human labour limits the ability to clinically control events when these mechanisms malfunction. Successful vaginal delivery requires strong contractions enabling the fetal head to dilate the cervix, separated by periods of relaxation permitting replenishment of placental blood flow [1] , [2] . A plateau phase is a particularly prominent feature of the action potential (AP) in human uterine smooth muscle (myometrium) [3] , [4] ; however, the ionic conductances responsible for determining the amplitude, duration and rapid repolarization of the plateau, to achieve relaxation between contractions, are unknown. The AP in cardiac muscle also has a prominent plateau component and the heart contracts forcefully during systole and then relaxes to permit refilling. The human ether-a-go-go-related gene (hERG1) potassium channel, I kr , plays an important role in repolarization of the prominent plateau of the cardiac AP and hence in determining AP, contraction and diastolic durations [5] . We hypothesized that hERG might play a role in regulating human uterine contractions. Potassium passes through the hERG α-pore-forming subunit and this is negatively regulated by a β-ancillary subunit [6] , [7] . The level of β-subunit protein increases in late pregnancy in mouse uterus [8] but the situation in labour has not been addressed. hERG has been identified in a range of smooth muscle tissues and pharmacological manipulation of its activity has an impact on contractile function [8] , [9] , [10] , [11] , [12] , [13] , [14] , [15] . Contractile function of uterine smooth muscle is impaired in obese women, who are more likely to experience failure to go into spontaneous labour and failure to progress through to vaginal delivery (18%) compared with normal weight controls (5%) [16] , [17] , [18] . This necessitates caesarean section, with the effects especially concentrated in the first stage of labour, when powerful contractions are required to dilate the cervix and move the fetus through the pelvis [16] , [17] , [18] . We now report that hERG proteins, both α-pore-forming and β-inhibitory subunits, are present in human myometrium in late pregnancy. The levels of β-inhibitory subunit are elevated in labour tissues and are associated with a decrease in hERG activity and an increase in AP and contraction duration. These changes that occurred in lean labouring women did not occur in obese labouring women and could explain the increased incidence of failure to progress in labour, necessitating caesarean delivery in obese women. hERG influences pregnant human uterine contractility To test whether hERG regulated AP duration we first recorded membrane potential and contraction simultaneously in strips of myometrium from lean women (body mass index (BMI) <30) at term before labour onset. We used dofetilide (1 μM) and E-4031 (1 μM) as they are selective for hERG blockade [19] and have been commonly used in smooth [8] , [9] , [10] , [11] , [12] , [13] , [14] , [15] and cardiac [5] muscles. Both blockers caused a striking prolongation of the AP plateau and contraction ( Fig. 1a ), from 0.9±0.2 to 2.8±0.2 min (a 2.9-fold increase, n =10, P <0.001, t -test; Fig. 1d ). This occurred without a depolarizing effect on resting membrane potential (−57±1 mV, Fig. 1a ). The hERG activator ICA-195574 (5 μM) [20] reduced contraction duration to 53±3% ( n =7, Fig. 2 ). 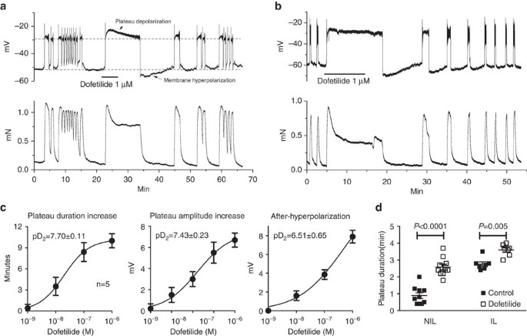Figure 1: hERG activity influences human uterine contractility. (a) Blockade of hERG with dofetilide (1 μM) prolonged the plateau phase of the AP (recorded using intracellular microelectrodes, upper trace) and contraction (lower trace) recorded simultaneously from a lower region strip, and (b) similar effects were recorded in a strip from the fundus (upper region) of the uterus. (c) Dofetilide induced a concentration-dependent increase in AP plateau duration, an increase in the level of plateau depolarization and an after-hyperpolarization between APs (n=5). (d) hERG block with dofetilide caused a greater prolongation of the AP plateau before (NIL) versus during labour (IL), effectively turning a NIL AP into an IL AP. Mean±s.e.m. andt-tests in (c). Figure 1: hERG activity influences human uterine contractility. ( a ) Blockade of hERG with dofetilide (1 μM) prolonged the plateau phase of the AP (recorded using intracellular microelectrodes, upper trace) and contraction (lower trace) recorded simultaneously from a lower region strip, and ( b ) similar effects were recorded in a strip from the fundus (upper region) of the uterus. ( c ) Dofetilide induced a concentration-dependent increase in AP plateau duration, an increase in the level of plateau depolarization and an after-hyperpolarization between APs ( n =5). ( d ) hERG block with dofetilide caused a greater prolongation of the AP plateau before (NIL) versus during labour (IL), effectively turning a NIL AP into an IL AP. Mean±s.e.m. and t -tests in ( c ). 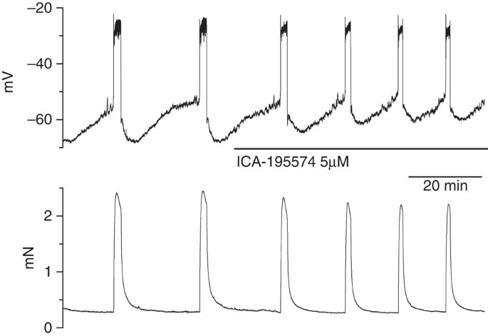Figure 2: Reduction in plateau duration by activation of hERG. Action potential plateau, recorded with an intracellular microelectrode, and contraction durations were reduced in the presence of the hERG activator ICA-195574. Full size image Figure 2: Reduction in plateau duration by activation of hERG. Action potential plateau, recorded with an intracellular microelectrode, and contraction durations were reduced in the presence of the hERG activator ICA-195574. Full size image Myometrium from the upper region (fundus) of the uterus was obtained from four women undergoing hysterectomy following caesarean delivery, and dofetilide prolonged the AP and contraction duration in a manner indistinguishable from its effects in the lower segment ( Fig. 1b ). The concentration dependence of dofetilide was tested using 20-min applications per dose in tissues from five women. There was a concentration-dependent increase in plateau duration (−log concentration required to induce a half-maximal response (pD 2 )=7.70±0.11), a more depolarized level of the AP plateau (pD 2 =7.43±0.23) and an after-hyperpolarization more negative than that observed basally (pD 2 =6.51±0.65; Fig. 1a,c ). Recovery from the after-hyperpolarization resulted in a prolongation of the time until the next AP from 6.8±1.4 min basally to 18.7±1.5 min in dofetilide ( P <0.0001, n =5, t -test). We acutely isolated myometrial cells from the same tissue samples and used whole-cell patch clamp techniques to interrogate the cells for hERG channel activity. The hERG current had a maximum amplitude of 3.6±0.4 pA pF −1 ( n =11; Fig. 3a,c ) and was blocked by dofetilide and E-4031 ( Fig. 3b,c ). Current was restored to ~70% upon washout of dofetilide for 20 min. The hERG current decayed with an exponential time course whose time constant displayed voltage dependence in which the time constant changed e-fold per 73 mV ( Fig. 3d , P <0.0001, F-test). These data are consistent with a mechanism by which, before labour, the depolarization during the AP activates hERG that shortens the duration of the plateau and its associated contraction, thereby facilitating quiescence. 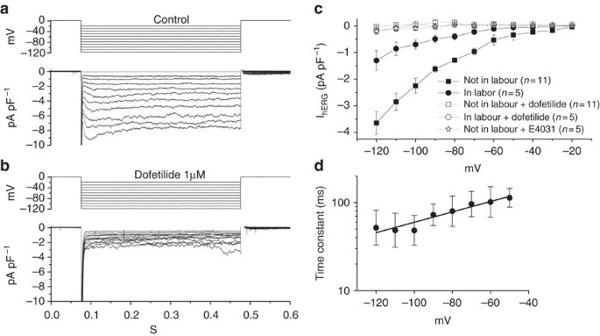Figure 3: hERG currents in isolated human myometrial cells. (a) In patch clamp of single isolated myometrial cells, following depolarization to 0 mV, in 140 mM extracellular K+solution, progressive step repolarizations to −120 mV evoked currents (b) that were blocked by dofetilide, indicating hERG. (c) hERG current was reduced to one-third in labour and blocked by dofetilide 1 μM and E-4031 1 μM.n=number of women tested, mean±s.e.m. (d) The voltage dependence of the time constant of deactivation changed e-fold per 73 mV (further analysis of data inanot in labour;P<0.0001, F-test). Figure 3: hERG currents in isolated human myometrial cells. ( a ) In patch clamp of single isolated myometrial cells, following depolarization to 0 mV, in 140 mM extracellular K + solution, progressive step repolarizations to −120 mV evoked currents ( b ) that were blocked by dofetilide, indicating hERG. ( c ) hERG current was reduced to one-third in labour and blocked by dofetilide 1 μM and E-4031 1 μM. n =number of women tested, mean±s.e.m. ( d ) The voltage dependence of the time constant of deactivation changed e-fold per 73 mV (further analysis of data in a not in labour; P <0.0001, F-test). Full size image Reduced hERG activity in the transition into normal labour We then asked whether changes in hERG function might contribute to the stronger, more co-ordinated contractions at the time of labour in lean women. In in-labour (IL) tissues dofetilide increased AP duration from 2.8±0.1 to 3.6±0.1 min ( P =0.005, n =7, t -test; Fig. 1d ), an increase of only 1.3-fold, and the maximum hERG current in single cells was reduced to 1.3±0.4 pA pF −1 ( Fig. 3c ). hERG (KCNH2) α-pore-forming subunit protein was detected in human myometrium using western blot analysis ( Fig. 4a ). The plasma membrane-inserted glycosylated 155-kDa form ( Fig. 4c ) and the endoplasmic reticulum-stored poorly glycosylated 135-kDa form ( Fig. 4d ) were identified and these bands were not observed in the presence of antibody-blocking peptide ( Fig. 4a ). hERG α-subunit protein levels were unchanged IL ( n =10) compared with not in labour (NIL; n =10, Fig. 4c ). Similarly, hERG α subunit mRNA did not differ IL versus NIL ( Fig. 4f ). 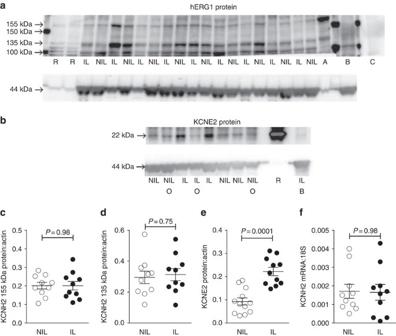Figure 4: hERG α- and β-subunit protein levels in human myometrium. (a) Western blots showing plasma membrane-inserted glycosylated 155-kDa and poorly glycosylated 135-kDa forms of hERG (upper trace) and α-actin 44-kDa (lower trace, loading control) in myometrium from lean women. R, rat heart; IL, in labour and NIL, not in labour myometrium; A, human adipose tissue-positive control; B blocking protein; C, antibody only. (b) KCNE2 β-subunit 22 kDa (upper trace). O, obesity. (c) Levels of pore-forming hERG α-subunit (KCNH2) 155 kDa (d) and 135 kDa were not different before (NIL) versus during labour (IL). (e) KCNE2 was significantly increased IL (Mean±s.e.m.,t-test). (f) Using qPCR, hERG α-subunit mRNA was not different NIL versus IL (ΔΔCtmethod followed by mean±s.e.m. andt-test). Figure 4: hERG α- and β-subunit protein levels in human myometrium. ( a ) Western blots showing plasma membrane-inserted glycosylated 155-kDa and poorly glycosylated 135-kDa forms of hERG (upper trace) and α-actin 44-kDa (lower trace, loading control) in myometrium from lean women. R, rat heart; IL, in labour and NIL, not in labour myometrium; A, human adipose tissue-positive control; B blocking protein; C, antibody only. ( b ) KCNE2 β-subunit 22 kDa (upper trace). O, obesity. ( c ) Levels of pore-forming hERG α-subunit (KCNH2) 155 kDa ( d ) and 135 kDa were not different before (NIL) versus during labour (IL). ( e ) KCNE2 was significantly increased IL (Mean±s.e.m., t -test). ( f ) Using qPCR, hERG α-subunit mRNA was not different NIL versus IL (ΔΔ C t method followed by mean±s.e.m. and t -test). Full size image Expression of β-auxiliary inhibitory subunit (KCNE2) protein was significantly enhanced IL versus NIL ( P =0.0001, Fig. 4b,e , t -test). The β-auxiliary subunit reduces current flow through the α-subunit of the hERG channel [6] , [7] , and its increase in the IL samples explains the suppression of hERG current and consequent prolongation of the AP plateau and contraction in labour. These data demonstrate that hERG contributes to suppression of uterine contractile strength before labour and this effect is reduced in labour in lean women, facilitating the strong contractions required for vaginal delivery. hERG effectiveness is increased as BMI increases Women with elevated BMI are more likely to have longer pregnancies, necessitating induction of labour [16] , [17] , [18] . Here we asked whether inappropriate hERG function in late pregnancy could contribute to this effect of obesity. We used the dofetilide-induced increase in AP plateau duration as a measure of hERG activity and plotted this against BMI. In tissues from women at term but NIL there was a strong positive correlation between dofetilide-induced increase in AP plateau duration and BMI. BMI explained 89% of the variance in plateau duration evoked by dofetilide ( r 2 =0.89, P <0.0001, least products regression, Fig. 5a ). Importantly, and consistent with this, hERG current density in isolated cells increased as BMI increased ( r 2 =0.59, P =0.001, least products regression, Fig. 5b ). 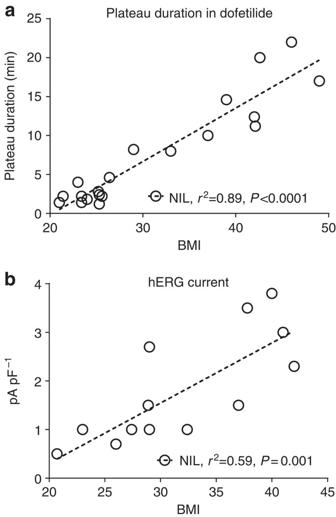Figure 5: BMI positively associated with increased hERG function in human myometrium. (a) The increase in plateau duration by dofetilide at term NIL was tightly correlated with increasing BMI. (b) hERG current was similarly increased with increasing BMI. Least products regression used. Figure 5: BMI positively associated with increased hERG function in human myometrium. ( a ) The increase in plateau duration by dofetilide at term NIL was tightly correlated with increasing BMI. ( b ) hERG current was similarly increased with increasing BMI. Least products regression used. Full size image This functional effect of elevated BMI was supported by a marked increase in hERG α-subunit protein ( r 2 =0.62, P <0.0001, least products regression, Fig. 6a ) and a decrease in inhibitory KCNE2 protein expression ( r 2 =0.33, P =0.004, Fig. 6b ) with increasing BMI. The reduction in β-subunit and increase in hERG expression with increasing BMI is consistent with greater hERG activity, which would shorten AP plateau and contraction duration, thus diminishing the prospects for the development of strong uterine contractions in women with an elevated BMI. 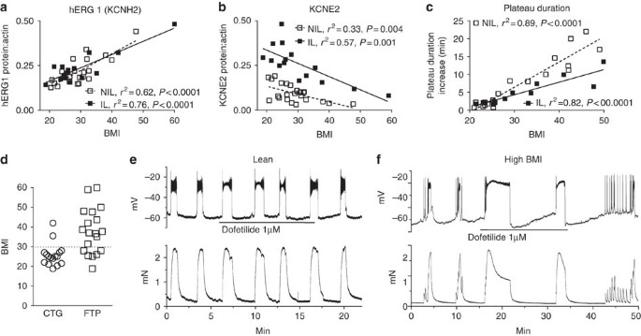Figure 6: hERG activity in myometrium persists in labour in obese women. (a) hERG 155 kDa protein increased with BMI in a similar manner before (NIL) and during labour (IL). (b) While KCNE2 protein was increased IL in lean tissue, this increase failed to occur as BMI increased. (c) The ability of dofetilide to increase AP plateau duration increased, indicating greater hERG and suppression of the AP and contraction with increasing BMI. Least products regression used. (d) All but two women with BMI >30 failure to progress in labour, while fetal distress (measured with the help of cardiotocography, CTG) necessitated caesarean delivery in 13 of 19 lean. (e) Examples showing that dofetilide was less effective in tissue from lean women IL compared with (f) tissue from obese women (membrane potential recorded from tissue strips using intracellular microelectrodes, upper traces, simultaneously with contraction, lower traces). Figure 6: hERG activity in myometrium persists in labour in obese women. ( a ) hERG 155 kDa protein increased with BMI in a similar manner before (NIL) and during labour (IL). ( b ) While KCNE2 protein was increased IL in lean tissue, this increase failed to occur as BMI increased. ( c ) The ability of dofetilide to increase AP plateau duration increased, indicating greater hERG and suppression of the AP and contraction with increasing BMI. Least products regression used. ( d ) All but two women with BMI >30 failure to progress in labour, while fetal distress (measured with the help of cardiotocography, CTG) necessitated caesarean delivery in 13 of 19 lean. ( e ) Examples showing that dofetilide was less effective in tissue from lean women IL compared with ( f ) tissue from obese women (membrane potential recorded from tissue strips using intracellular microelectrodes, upper traces, simultaneously with contraction, lower traces). Full size image Uterine hERG activity persists in labouring obese women In labour, women with a higher BMI more often fail to progress through to vaginal delivery, necessitating caesarean section [16] , [17] . The dramatic effects of BMI on hERG activity and on AP and contraction duration before labour prompted the critical question: does this suppressive effect of hERG persist in labour and account for the failure to progress in labour in obesity? In our cohort of lean women, BMI <30, the reason for caesarean delivery was non-reassuring fetal welfare status (indicated with the help of cardiotocography) in 13 of 19 women, with failure to progress in only 6 of the 19 women ( Fig. 6d ). In contrast, for women with BMI >30, failure to progress occurred in 14 of 16 cases ( Fig. 6d ). Dofetilide had only a modest effect on AP and contraction duration in myometrial strips from lean women IL ( Fig. 6e ) but was more effective in strips from obese women ( Fig. 6f ). The increase in AP plateau duration by dofetilide in IL tissues increased progressively as BMI increased ( r 2 =0.82, P <0.0001, least products regression, Fig. 6c ). While the increase in α subunit of hERG with BMI was similar in IL ( r 2 =0.76, P <0.0001) and NIL tissues ( r 2 =0.62, P <0.0001, least products regression, Fig. 6a ), levels of β-subunit protein declined as BMI increased to a greater extent in IL samples ( r 2 =0.57, P =0.001, least products regression, Fig. 6b ). Thus, for larger BMI there is little difference in levels of β-subunit protein between IL and NIL. Since the β-subunit suppresses hERG current, its increase in lean labour removes the hERG termination of the AP and contraction permitting longer and likely more effective contractions, thereby facilitating vaginal delivery. Conversely, the strong decrease in β-subunit protein levels in women with elevated BMI effectively means that the myometrium does not fully transform into a labouring phenotype (hERG remains strong and contractions remain weak), and this provides a mechanistic explanation for the failure to progress in labour in many women with increasing BMI. Here we provide compelling evidence that hERG plays a significant role in the relative quiescence of the uterus before labour, essential for development of the fetus to maturity. This is achieved by the ability of hERG to shorten the plateau phase of the AP, providing insufficient time for the development of a large contraction in human myometrium. The resulting contraction is short and weak. The transition of the myometrium into a labouring phenotype is accompanied by changes in hERG activity, whereby hERG-associated suppression of the uterine AP is markedly reduced. In fact, when we blocked hERG in not in labour tissues, the AP duration was transformed into one with a prolonged labour-like duration (see Fig. 1d ). In contrast, during labour, APs and contractions are prolonged and hERG blockade is much reduced. The labour-associated reduction in hERG effectiveness occurs despite maintained levels of hERG α-pore-forming subunit protein and mRNA. Rather, there is a marked increase in β-auxiliary subunit expression, which suppresses hERG current [6] . Blockade of hERG with dofetilide or E-4031 results in depolarization in rat stomach [12] , bovine epididymal [11] and opossum oesophageal [9] smooth muscles. This likely accounts for the increase in contraction frequency created by hERG blockade in most smooth muscle tissues studied [8] , [10] , [14] . In contrast, human myometrium was hyperpolarized between APs in the presence of dofetilide, which was accompanied by a decrease in contraction frequency. This hyperpolarization is likely a consequence of the prolonged nature of the human uterine AP plateau in the presence of hERG blockers, rather than as a direct result of hERG blockade. This interpretation arises from our previous finding that application of prostaglandin F 2α to human myometrial strips results in prolongation of the AP plateau and an after-hyperpolarization between APs, reminiscent of the consequences of dofetilide application observed here. We established that the prostaglandin effect is because of an increase in Na/K ATPase activity as a result of AP plateau lengthening [21] . Thus, understandable differences in ion channel type and density and physiological consequences in terms of contraction duration and frequency occur in human uterine versus other smooth muscles [2] . Many smooth muscle tissues display plateau-like electrical activity, which dictates the amplitude and duration of contraction [22] , [23] , [24] , [25] , and this includes the circular muscle layer of the mouse myometrium [24] . While the level of the plateau in many cases is close to that observed in human myometrium, −25 to −30 mV, a striking feature of the AP plateau in human myometrium is the rapidity of repolarization. Block of hERG in guinea pig gall bladder increases the duration of a proportion of pacemaker depolarizations permitting an increase in the number of superimposed spike APs [14] . In human jejunum, E4031 increases the amplitude of all pacemaker depolarizations, again increasing the number of spike APs [10] . Taken together, the use of hERG blockers in the present study provides insights into the unique nature of the plateau-AP in human uterus, demonstrates an important role for hERG potassium channels and provides an impetus for further study. The voltage dependence of the rate of deactivation of hERG current in smooth muscle cells is much weaker than that of hERG in cardiomyocytes [13] , [15] , [26] . Furthermore, in mouse myometrium the voltage dependence appears weaker in late pregnancy compared with non-pregnant tissue [8] . Our results show a weak voltage dependence for myometrium of women at term, consistent with the earlier studies in late pregnant mouse myometrium [8] . Activation of protein kinase A (PKA) increases hERG protein phosphorylation, which facilitates hERG incorporation into the plasma membrane [27] . PKA may also influence activity of the inhibitory β-subunit [28] . Within the myometrium, cAMP activation of PKA pathways is involved in maintaining relaxation during pregnancy, and components of PKA signalling are downregulated in human labour [29] permitting strong contractions. It remains to be determined whether regulation of hERG activity in the transition into human labour involves the cAMP/PKA signalling system. Obesity is an increasing medical problem within the population in general and, consequently, is increasing in the pregnant population. Obesity is largely responsible for the recent increasing need for caesarean delivery, which increases maternal and neonatal morbidity and can predispose to problems for future pregnancies [30] , [31] . The hERG β-subunit is upregulated by oestrogen [32] , and the oestrogen profile can be dysfunctional in high BMI pregnancies [33] . Obesity is associated with increased circulating levels of cholesterol and leptin [34] . Cholesterol levels are higher in caveoli [35] , the location of hERG α- and β-subunit insertions [36] . Direct interaction may occur between membrane lipids and amino acids in membrane-traversing domains of ion channel proteins [37] , and hERG channel kinetics are sensitive to the cholesterol content of the plasma membrane [36] . Disruption of membrane cholesterol suppresses human and rat uterine contractions [38] . Leptin is also increased in obesity and during pregnancy [39] , and leptin [40] and the adipokine apelin [41] also suppress human uterine contractions. The role of these factors in regulating hERG α- and β-subunits in human myometrium warrants investigation. Here we demonstrate for the first time the presence of hERG protein and β-ancillary subunit protein in human myometrium in late pregnancy and labour. Our results demonstrate the dynamic contribution of hERG channels, and the β-subunit in particular, to uterine smooth muscle function in the progression into labour. Importantly, we show that hERG is present and influences contractility, not only in the lower segment but also within the main fundus region of the uterus. Effectively, blockade of hERG by dofetilide transforms the pre-labour myometrium into the labouring phenotype ( Fig. 1d ). Significantly, our results draw together a strong link between obesity and hERG function in human myometrium. Thus, our data present compelling evidence implicating hERG channels in the established clinical problem of the rising incidence of caesarean delivery in obesity and provide a focus for further investigation. We provide a solid mechanism towards understanding the poor labour outcomes in obese women. Studies were approved by the Royal Women’s Hospital Research Ethics Committee, and the Hunter and New England Area Research Committee, adhering to the guidelines of the Declaration of Helsinki. Participants gave informed written consent for collection of myometrial samples before surgery and tissue collection. BMI was obtained at first hospital visit. Women with singleton pregnancies undergoing term (37–40 weeks gestation) elective caesarean delivery with no signs of labour formed the NIL cohort ( n =43), while women undergoing term emergency caesarean section following the spontaneous establishment of labour formed the IL cohort ( n =27). Infection, hypertension and diabetes were exclusion criteria. Clinical indications for elective NIL caesarean delivery were previous caesarean section, 3rd/4th degree tear and breech presentation, while clinical indications for emergency IL caesarean section were non-reassuring fetal welfare status or failure to progress in labour. Following delivery of the placenta, all women were administered 10 units of oxytocin (syntocinon) directly into an intravenous line as part of standard care for the prevention of post-partum haemorrhage. Myometrial biopsies were excised 3–5 min after administration of oxytocin; thus, all samples were briefly exposed to oxytocin. Myometrial samples (5 × 5 × 10 mm) from the lower uterine segment were studied in most cases. However, four women underwent hysterectomy following caesarean delivery and fundus tissue was studied. A portion of the sample was immediately frozen in liquid nitrogen for subsequent protein analysis, while the remaining tissue was immediately taken to the laboratory and electrophysiology and contraction studies were commenced within 1 h. Strip electrophysiology and contraction Membrane potential was recorded from smooth muscle cells in strips of tissue (3 × 1 × 0.5 mm), using glass intracellular microelectrodes filled with 1 M KCl (resistances ~100 MΩ) to impale a single smooth muscle cell within the strip, and tension was recorded simultaneously (force transducer, AE801, SensoNor, Horton, Norway) [21] . The microelectrode was connected to an Axoclamp 2B amplifier (Axon Instruments, CA, USA), low-pass-filtered at 3 kHz and digitized at 1 kHz (Digidata 1440A, Molecular Devices, CA, USA). Strips were set at 0.2mN basal tension and continuously superfused at 3 ml min −1 and 36 °C with physiological salt solution (PSS) containing the following (in mM): NaCl 120, KCl 5, NaHCO 3 25, KH 2 PO 4 1, MgSO 4 1.2, CaCl 2 2.5, glucose 11, gassed with 95% O 2 , 5% CO 2 , pH 7.4. Concentration response curves to dofetilide were fitted to a sigmoid curve, using the least-squares method and pD 2 (−log EC 50 ) was calculated (GraphPad Prism). Patch clamp Single smooth muscle cells were isolated (2 mg ml −1 type I collagenase, 2 mg ml −1 trypsin inhibitor, 1 mg ml −1 fatty acid-free albumin at 37 °C for 50 min) and studied within 6 h. The cells were voltage-clamped using whole cell or nystatin-perforated patches (Axopatch 200 and Digidata 1322A, pClamp 9). Cells were superfused with PSS (in mM): NaCl 137, NaHCO 3 4, NaH 2 PO 4 0.3, KCl 5.4, KH 2 PO 4 0.44, MgCl 2 0.5, MgSO 4 4, glucose 5.6, HEPES 10, CaCl 2 1.3, at pH 7.4 and 22 °C. Patch electrode solution contained the following (in mM): KCl 130, MgCl 2 1.2, ATP 3, EGTA 5, HEPES 10. To enhance K + currents, the PSS contained (mM) the following: KCl 140, MgCl 2 1, HEPES 10, glucose 10, CaCl 2 0.1 immediately before testing. Cells were held at 0 mV and stepped in 10-mV increments to −120 mV (refs 8 , 9 ). Western blotting Protein analysis was performed as previously outlined [42] . Rabbit anti-K v 11.1 (hERG) (APC-109, 1:2,000 dilution, Alomone Laboratories, Israel) and rabbit anti-KCNE2 (APC-054, 1:200 dilution, Alomone Laboratories) were applied in the presence or absence of blocking peptide (2 μg per 1 μg antibody). Protein was expressed relative to α-smooth muscle actin and analysed using t -tests with unequal variance. Full-length images of immunoblots are shown in Supplementary Figs 1 and 2 . mRNA determination Total RNA was extracted and purified from NIL ( n =10) and IL ( n =10) samples using the trizol-chloroform method and treated with deoxyribonuclease to remove contaminating genomic DNA. RNA was quantified and 1 μg reverse-transcribed with random hexamers using Superscript III reverse transcriptase (Life Technologies, Australia). The primers for KCNH2 (Hs00542479_g1, Invitrogen) and 18s rRNA (4319413E, Invitrogen) were labelled with FAM and VIC, respectively. Quantitative PCR was performed using a TaqMan universal master mix and monitored during cycling in an ABI PRISM 7500 sequence detector (Applied Biosystems). The cycling conditions were 50 °C for 2 min, 95 °C for 10 min and 40 cycles of 95 °C for 15 s, 60 °C for 1 min. The cycle at which fluorescence reached a set threshold (cycle threshold) was used for quantitative analyses. Cycle threshold in each assay was set at a level at which the exponential increase in amplicon abundance was approximately parallel between all samples. mRNA abundance was expressed relative to 18S rRNA and analysed using the ΔΔ C t method. Reagents Stock solutions of blockers and activators of hERG channels were prepared in DMSO at × 1,000 concentration or dH 2 O as appropriate. The hERG blockers dofetilide and E-4031, activators PD-118057, NS1643 and ICA-195574, dimethylsulphoxide (DMSO) and all solution reagents were purchased from Sigma-Aldrich (St Louis, USA). DMSO 1:1,000 dilution was tested for the appropriate time exposure in every tissue. There was no detectable effect of DMSO on activity in whole tissues or isolated single smooth muscle cells. Statistical analysis Data were analysed using GraphPad Prism and GraphPad InStat (GraphPad Software Inc., San Diego, CA, USA). For all data sets, equality of s.d.’s and Gaussion distribution, using the Kolmogorov/Smirnov method, were tested. Data are expressed as the mean and s.e.m. Throughout, n represents the number of women studied and P <0.05 was accepted as statistically significant. Experimenters were blinded to the clinical status of the women (NIL, IL, BMI) and the status was provided by Dr P Sheehan at a stage in the analysis when it was required. For electrophysiology and contractility studies, correlation between dofetilide-induced plateau lengthening and BMI was determined using least products regression. Analyses of variance were used to compare between NIL versus IL and to test hERG currents and dofetilide effects versus BMI, with Bonferonni post hoc testing. Unpaired or paired Student’s t -tests were used for testing differences. How to cite this article: Parkington, H. C. et al . Diminished hERG K + channel activity facilitates strong human labour contractions but is dysregulated in obese women. Nat. Commun. 5:4108 doi: 10.1038/ncomms5108 (2014).